A hydrophobic Cu/Cu2O sheet catalyst for selective electroreduction of CO to ethanol Electrocatalytic reduction of carbon monoxide into fuels or chemicals with two or more carbons is very attractive due to their high energy density and economic value. Herein we demonstrate the synthesis of a hydrophobic Cu/Cu 2 O sheet catalyst with hydrophobic n-butylamine layer and its application in CO electroreduction. The CO reduction on this catalyst produces two or more carbon products with a Faradaic efficiency of 93.5% and partial current density of 151 mA cm −2 at the potential of −0.70 V versus a reversible hydrogen electrode. A Faradaic efficiency of 68.8% and partial current density of 111 mA cm −2 for ethanol were reached, which is very high in comparison to all previous reports of CO 2 /CO electroreduction with a total current density higher than 10 mA cm −2 . The as-prepared catalyst also showed impressive stability that the activity and selectivity for two or more carbon products could remain even after 100 operating hours. This work opens a way for efficient electrocatalytic conversion of CO 2 /CO to liquid fuels. Electrochemical CO 2 reduction reaction (CO 2 RR) to energy-efficient fuels and chemicals could be a solution to relieve the dependency on fossil fuel and mitigate the greenhouse gas effect [1] , [2] , [3] , [4] . Production of single carbon products is relatively simple, e.g., the CO 2 RR to CO is currently being developed for commercial applications [5] , [6] , [7] , [8] . Products with two or more carbons (C 2+ products), such as ethylene, acetic acid and ethanol, are useful chemicals or fuels with obvious economic value. Thus, efficient CO 2 RR to C 2+ products is of great importance. Cu-based catalysts have been shown to be efficient for converting CO 2 into C 2+ products with appreciable selectivity [9] , [10] , [11] . However, research work still needs to focus on reducing the cathodic overpotential and further improving C 2+ product selectivity [12] , [13] . CO is known as a key reaction intermediate on the pathway to C 2+ compounds. The CO reduction reaction (CORR) has received increased attention and showed significant promise since recent progress demonstrated high-rate CORR operation, which raises the attractive prospect of dividing the total conversion of CO 2 into discrete steps with CO as the intermediate feedstock [14] , [15] , [16] . Some approaches for CORR have shown improved selectivity to C 2+ [15] , [17] . For example, CORR to ethylene has been reported with Faradaic efficiency (FE) of up to 52.7% through optimization of cathode structure to facilitate CO diffusion at the surface of the electrode and Cu catalysts [18] . By constraining CO coverage on copper, an ethylene FE of 72% and a partial current density of >800 mA cm −2 could be achieved [19] . Recently, ethylene could be formed with FE of 87% ± 3% through the introduction of a polymer that is entrained on the electrode surface [14] . It can be seen that ethylene could be generated with both high FE and high molar production. By contrast, there are few studies on the ethanol formation from CORR. Ethanol is of particular interest as it has high energy density, high market price and consistent global demand [20] . 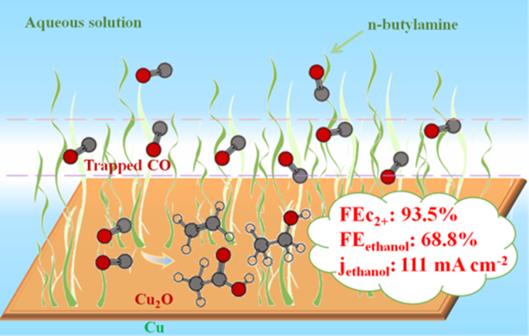Fig. 1: Schematic illustration of the hydrophobic Cu/Cu2O catalyst designed for CORR. The n-butylamine on the Cu/Cu2O surface is used to trap the CO molecules. However, for a total current density higher than 10 mA cm −2 , the FE for ethanol from CORR process still needs to be further improved (Supplementary Table 1 ) [21] . Also very often the catalysts suffered from poor stability [22] . Exploration of catalysts with high catalytic activity, selectivity and stability for ethanol in CORR process still remains a challenging task [23] , [24] . In this work, we construct a stable Cu-based catalyst with high efficiency for ethanol formation in CORR process. Previous reports indicated that surface structure of electrocatalysts has great effect on the performance for CO 2 /CO electroreduction [25] , [26] . Preoxidation of Cu greatly boosted its intrinsic catalytic properties toward C 2+ formation in CO 2 RR [27] . Computational studies suggested that Cu + can function synergistically with Cu 0 to promote C 2 production because of the easier CO 2 activation and C-C coupling [28] . Though several approaches were employed to stabilize the Cu + species, the active Cu + species are still very prone to being reduced under CO 2 RR conditions [29] . And for CORR, there are very few studies on whether oxides on the catalyst surface play a crucial role in selectivity improvement. On the other hand, hydrophobicity was proposed as one of the governing factors in CO 2 /CO reduction selectivity [4] , [18] . The above investigations inspire us to design Cu/Cu 2 O catalyst by adopting a hydrophobic strategy and study the performance of C 2+ products especially ethanol formation in CORR. Here we report a facile one-pot synthesis method to synthesize hydrophobic Cu/Cu 2 O catalyst for CO electroreduction. Cu/Cu 2 O coated with n-butylamine was obtained with tunable hydrophobicity. As shown in Fig. 1 , the resulted catalyst with appropriate amount of n-butylamine layer offering suitable hydrophobicity would reduce the affinity of water to the electrode and promote the diffusion and affinity of CO to the electrode interface (see Supplementary Tables 2 - 3 for the diffusion coefficients and solubility of CO in water and n-butylamine), thus H 2 evolution on the surface could be suppressed to some extent in CO-saturated electrolyte. At −0.7 V vs reversible hydrogen electrode (RHE), the FE of C 2+ products could reach 93.5% with a current density of 151 mA cm −2 , including 68.8% of FE for ethanol, 19.6% for ethylene and 5.1% for acetic acid. The FE of ethanol is very high in comparison to all previous reports of CO 2 /CO electroreduction, as can be known from Supplementary Table 1 , which could benefit from both the increased CO concentration at the hydrophobic surface and the exposure of Cu 2 O (111) on the surface. Fig. 1: Schematic illustration of the hydrophobic Cu/Cu 2 O catalyst designed for CORR. The n-butylamine on the Cu/Cu 2 O surface is used to trap the CO molecules. Full size image Synthesis and characterization of hydrophobic Cu/Cu 2 O catalyst The Cu/Cu 2 O catalyst was prepared by one-pot synthesis method through chemical reduction. Glucose aqueous solution with desired amount of polyvinyl pyrrolidone (PVP)/hexadecyl trimethyl ammonium bromide (CTAB) and n-butylamine was added dropwise into the Cu(acac) 2 -N,N-dimethyl formamide (DMF) solution. Then this solution was sealed and heated at 160 °C for 10 h. The Cu/Cu 2 O catalyst (denoted as Cu/Cu 2 O-A) was obtained after cooling down and washing. Scanning electron microscope (SEM) showed the Cu/Cu 2 O mainly exhibited sheet morphology (Fig. 2 a, d). The corresponding lattice distances of Cu and Cu 2 O were 0.180 nm and 0.247 nm, respectively, observed by the high-resolution transmission electron microscopy (HRTEM) (Fig. 2 b, c, e, f), indicating the co-existence of Cu and Cu 2 O in the as-prepared catalyst. The powder X-ray diffraction measurement (XRD) showed the characteristic peaks of metallic Cu (Supplementary Fig. 1a ). The crystal feature of Cu 2 O could hardly be observed by XRD due to the low loading (1.74 wt% according to the Nitrogen-Oxygen analyzer). Fig. 2: SEM and TEM images for Cu/Cu 2 O-A. 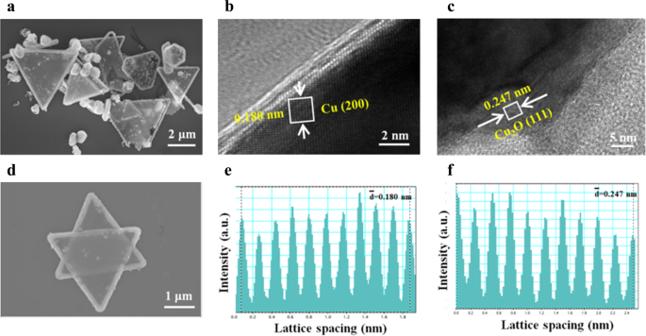Fig. 2: SEM and TEM images for Cu/Cu2O-A. a,dSEM,b,cTEM ande,fIntensity profiles measured from the regions marked by the white squares in images b and c, respectively. a , d SEM, b , c TEM and e , f Intensity profiles measured from the regions marked by the white squares in images b and c, respectively. Full size image X-ray photoelectron spectroscopy (XPS) was conducted to investigate the surface chemical composition and elemental valence states of the Cu/Cu 2 O-A catalyst (Fig. 3 ). The XPS spectrum revealed peaks of Cu species at 952.4 eV (Cu 2p 1/2 ) and 932.6 eV (Cu 2p 3/2 ) (Fig. 3a ). Auger electron spectroscopy (AES) was employed to further evidence that the signal was mainly derived from Cu 2 O [30] , [31] (Fig. 3b ). As XPS has limitations with regard to probe depth (detection depth often less than 10 nm), we etched the Cu/Cu 2 O-A with 5 nm and 10 nm depths. After etching, it showed the characteristic peaks of Cu 0 , indicating the Cu was covered with Cu 2 O on the surface (Fig. 3b ). In addition, the n-butylamine layer on the surface of Cu/Cu 2 O-A catalyst was also confirmed by XPS (Fig. 3 c, d). The high-resolution N 1 s spectra showed a peak at 398.8 eV (N 1 s ), which belongs to the n-butylamine coated on the surface. Control spectra had been carried out to prove the N species in N 1s spectra is from n-butylamine, not from the possible impurities DMF or CTAB (Supplementary Fig. 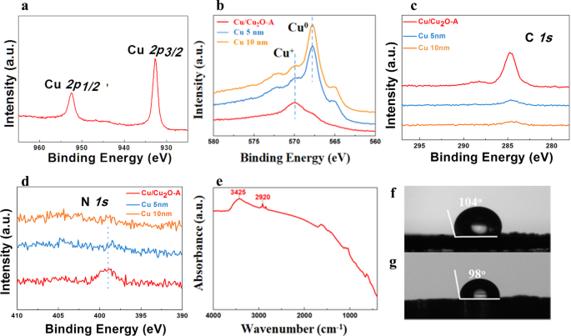Fig. 3: Characterization of the Cu/Cu2O-A. aCu2pXPS spectrum of the as prepared hydrophobic Cu/Cu2O-A catalyst.bCuLMM,chigh-resolution C1sspectra, anddhigh-resolution N1sspectra of Cu/Cu2O-A (red), Cu 5 nm (blue) and Cu 10 nm (orange) (Cu 5 nm refers to Cu/Cu2O-A catalyst etched with 5 nm depth; Cu 10 nm refers to Cu/Cu2O-A catalyst etched with 10 nm depth).eFT-IR of Cu/Cu2O-A. Images of the water contact angle of the as-prepared Cu/Cu2O-A catalystfand that after 100 h of CORR at −0.7 V vs RHEg. 1b ). Moreover, the strong infrared (IR) absorption bands at 3425 and 2920 cm −1 (Fig. 3e ) further suggested that n-butylamine covered the surface of Cu/Cu 2 O-A [32] , [33] . A water contact angle (CA) of 104° (Fig. 3f ) demonstrates that the n-butylamine-treated Cu/Cu 2 O electrode is impassible to the wetting and this falls into the regime of hydrophobicity of trapping gases [4] . The hydrophobic/hydrophilic property could be easily tuned by the amount of n-butylamine. Modification with larger amount of n-butylamine leads to highly hydrophobic surface of Cu/Cu 2 O catalyst (Supplementary Figs. 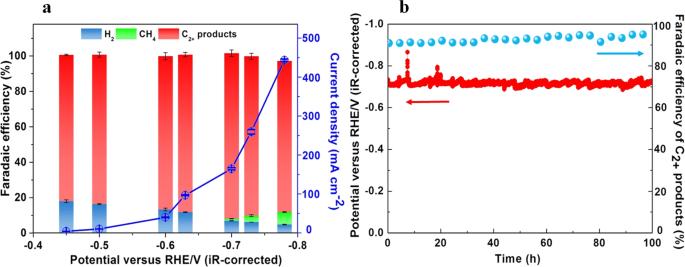Fig. 4: CO electroreduction performance of hydrophobic Cu/Cu2O-A. aTotal current density and Faradaic efficiencies for C1(green), C2products (red) and hydrogen (blue) obtained during CORR in 2.0 M KOH versus applied potential.bStability test over a span of 100 h of electrolysis at 164 mA cm−2in 2.0 M KOH. The loading of Cu/Cu2O-A is 2 mg cm−2. Error bars represent the standard deviations calculated from three independent measurements. 2 – 4 and Supplementary Table 4 ). Fig. 3: Characterization of the Cu/Cu 2 O-A. a Cu 2p XPS spectrum of the as prepared hydrophobic Cu/Cu 2 O-A catalyst. b Cu LMM , c high-resolution C 1 s spectra, and d high-resolution N 1 s spectra of Cu/Cu 2 O-A (red), Cu 5 nm (blue) and Cu 10 nm (orange) (Cu 5 nm refers to Cu/Cu 2 O-A catalyst etched with 5 nm depth; Cu 10 nm refers to Cu/Cu 2 O-A catalyst etched with 10 nm depth). e FT-IR of Cu/Cu 2 O-A. Images of the water contact angle of the as-prepared Cu/Cu 2 O-A catalyst f and that after 100 h of CORR at −0.7 V vs RHE g . Full size image To complement the results from XPS/XRD/HRTEM and the quantification of Cu 2 O phase by the Nitrogen-Oxygen analyzer, we have used X-ray absorption spectroscopy (XAS) to further investigate the Cu species. Unlike XPS (a surface-sensitive technique), XAS is inherently a bulk-sensitive technique and an average phenomenon accounting for all the Cu atoms in the sample. Supplementary Figs. 5a and 5b display the spectra of Cu K-edge X-ray absorption near edge structure (XANES) and extended X-ray absorption fine structure (EXAFS) for the Cu/Cu 2 O-A catalyst and the corresponding Cu standards. They both seem to indicate a high resemblance of the Cu/Cu 2 O-A catalyst with the metallic Cu. Given the nature of the technique, this is well in-line with the XPS Cu LMM Auger results showing that a thin Cu 2 O layer (1.74 wt%) covering the metallic Cu surface of the catalyst; under these circumstances, it is reasonable to assume that XAS is hard to detect the low amount of Cu 2 O localized selectively (in a thin layer) over the catalyst surface. This result also explained why it is hard to see the peaks derived from Cu 2 O in the XRD pattern. All the above results demonstrate that the as-prepared Cu/Cu 2 O-A consists of a metallic copper core with a Cu 2 O shell that is further covered by a layer of n-butylamine. The combination of the reducing agent and stabilizing agent was the key to successful synthesis of Cu/Cu 2 O-A. As the reducing agents, DMF and D- (+) –glucose reduced Cu (II) to Cu (0) or Cu (I). During this process, part of Cu (I) was protected by n-butylamine from further reduction to Cu (0) [31] , [34] . Meanwhile, n-butylamine was adsorbed on the surface to reduce surface energy and avoid aggregation. What’s more, the layer of n-butylamine acting as the stabilizing agent could restrain oxidation of Cu or Cu 2 O to offer good stability of the oxidation state of the catalyst, which would last 16 months without obvious change under ambient conditions (Supplementary Fig. 6 ). Electrocatalytic CORR performance The CORR performance tests were carried out at various potentials in a flow cell reactor, employing KOH as the electrolyte (Supplementary Fig. 7 ). Figure 4a shows that the as-prepared hydrophobic Cu/Cu 2 O-A offers good efficiency for CO reduction to C 2+ products. The maximum FE for C 2+ products reached as high as 93.5% in 2.0 M KOH at the potential of −0.7 V vs RHE. The FE of ethanol could reach 68.8% with a partial current density of 111 mA cm −2 at −0.7 V vs RHE. With the increasing of the applied overpotentials, the rapid growth of current densities indicated that the mass transfer resistance of CO was low. Fig. 4: CO electroreduction performance of hydrophobic Cu/Cu 2 O-A. a Total current density and Faradaic efficiencies for C 1 (green), C 2 products (red) and hydrogen (blue) obtained during CORR in 2.0 M KOH versus applied potential. b Stability test over a span of 100 h of electrolysis at 164 mA cm −2 in 2.0 M KOH. The loading of Cu/Cu 2 O-A is 2 mg cm −2 . Error bars represent the standard deviations calculated from three independent measurements. Full size image Moreover, the hydrophobic Cu/Cu 2 O-A showed a stable C 2 species FE for 100 h (Fig. 4b ). Impressively, even after 100 h of electroreduction reaction, the amount of Cu + on the catalyst surface was still the same as that in the virgin sample, reflecting the high stability of hydrophobic Cu/Cu 2 O-A and the protective effects of n-butylamine (Supplementary Figs. 8 - 10 ). What’s more, to ensure the repeatability, another two independent stability measurements were carried out under the same conditions and time duration (Supplementary Fig. 11 ). The water CA (98°) on the catalyst after 100 h of CORR at −0.7 V vs RHE was very close to that of the fresh one, indicating that the hydrophobic surface of Cu/Cu 2 O-A was well maintained during the CORR process (Fig. 3g ). XPS analysis and elemental analysis before and after the 100 h of electrolysis exhibited similar contents of C and N on the surface of the hydrophobic Cu/Cu 2 O-A, further confirming the well-maintenance of the hydrophobic butylamine layer on the surface (Supplementary Fig. 8 and Supplementary Table 4 ). The in-situ Raman spectra of the catalyst during the electroreduction with the laser excitation at 532 nm were obtained. At the applied potential of -1.77 V vs Ag/AgCl for 12 min, the characteristic peaks at 220 and 632 cm −1 for Cu 2 O retained, suggesting Cu + is persistent under electrocatalytic conditions (Supplementary Fig. 12 ). At the same time, due to the low polarity, CO tends to stay close to the hydrophobic tail of n-butylamine. Furthermore, reports have shown that the hydrophobic layer could trap gas to form an electrolyte-electrode-gas triple phase boundary [4] , [35] , [36] . Thus in this study we speculated that n-butylamine could act as a stabilizer for Cu + and form voids that trapped CO to offer an electrolyte-electrode-gas triple phase boundary, which might enhance the long-term stability of the Cu/Cu 2 O catalyst. To confirm that CO was the carbon source of C 2 products, we conducted the blank experiments using N 2 to replace CO in the electrolysis. The experiments showed that no product was formed in the electrolysis when using N 2 (Supplementary Fig. 13 ). To further verify that the product was derived from CO reduction, isotope labeled 13 CO experiment was conducted using Cu/Cu 2 O-A. From the mass spectra, we can observe 13 C signal for the main liquid product ethanol (Supplementary Fig. 14 ) and the main gas product ethylene (Supplementary Fig. 15 ), revealing that the C 2 products were derived from CO rather than other C-based chemicals in our reaction system. In order to reveal the role of the hydrophobicity on the high C 2+ FE and good stability of the Cu/Cu 2 O catalyst we further synthesized another two samples with different hydrophilicity and hydrophobicity denoted as Cu/Cu 2 O-S (highly hydrophobic) and Cu/Cu 2 O-H (hydrophilic) by adjusting the added amount of n-butylamine. Cu/Cu 2 O-S and Cu/Cu 2 O-H showed water CA of 130° and 50°, respectively (Supplementary Fig. 4 ). These two samples showed similar XRD patterns and FT-IR spectra with Cu/Cu 2 O-A but with different amount of n-butylamine on the surface (Supplementary Figs. 2 and 6 ). 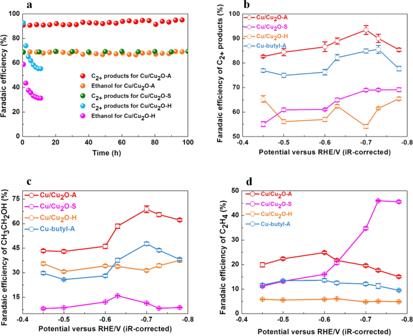Fig. 5: Faradaic efficiency of various products for Cu-based catalysts. aStability test of electrolysis in 2.0 M KOH for Cu/Cu2O-A, Cu/Cu2O-S and Cu/Cu2O-H.bFE of C2+products,cFE of ethanol, anddFE of ethylene for CO electroreduction on Cu/Cu2O-A (red), Cu/Cu2O-S (purple), Cu/Cu2O-H (orange) and Cu-butyl-A (blue). The loading of Cu/Cu2O-A is 2 mg cm−2. Error bars represent the standard deviations calculated from three independent measurements. Figure 5a shows the stability test of all of the three samples (Cu/Cu 2 O-A, Cu/Cu 2 O-S and Cu/Cu 2 O-H) over 100 h; while the data present in Fig. 5b-d for Cu/Cu 2 O-H were collected after 10 h when the performance was relatively stable. Cu/Cu 2 O-A, Cu/Cu 2 O-S and Cu/Cu 2 O-H with different hydrophobicity showed good FEs and current densities of C 2+ products, offering 93.5% (at −0.7 V), 69.1% (at −0.78 V) and 65.4% (at −0.78 V) FEs, respectively (Fig. 5b and Supplementary Figs. 16 and 17 ). While the hydrophobic Cu/Cu 2 O-A and Cu/Cu 2 O-S could give stable FEs of C 2+ products over 100 hours, hydrophilic Cu/Cu 2 O-H was quite unstable as the gas diffusion layer became flooded and then the activity quickly decreased during operation [35] , indicating the suitable hydrophobicity is vital for good stability (Fig. 5a and Supplementary Fig. 18 ). Both Cu/Cu 2 O-A and Cu/Cu 2 O-H showed high FEs of ethanol, reaching maximum value of 68.8% (at -0.7 V) and 37.6% (at -0.78 V) (Fig. 5c and Supplementary Fig. 17 ). Cu/Cu 2 O-S with the highest hydrophobicity, however, favors producing ethylene (46%) and shows quite low FE (8.3%) of ethanol at -0.73 V vs RHE (Fig. 5 c, d and Supplementary Fig. 17 ). At the same time, Cu/Cu 2 O-H showed much higher H 2 FE because its high hydrophilicity increases the affinity of water to the catalyst and thus decreases the number of the active sites for CORR (Supplementary Figs. 18 and 19 ). Therefore, a proper hydrophobicity can reduce the affinity of water to the electrode, enhance the stability and at the same time promote the diffusion of CO to the water-electrode interface, but too high hydrophobicity favors producing ethylene over ethanol, and too high hydrophilicity decreases the stability of the electrode. Fig. 5: Faradaic efficiency of various products for Cu-based catalysts. a Stability test of electrolysis in 2.0 M KOH for Cu/Cu 2 O-A, Cu/Cu 2 O-S and Cu/Cu 2 O-H. b FE of C 2+ products, c FE of ethanol, and d FE of ethylene for CO electroreduction on Cu/Cu 2 O-A (red), Cu/Cu 2 O-S (purple), Cu/Cu 2 O-H (orange) and Cu-butyl-A (blue). The loading of Cu/Cu 2 O-A is 2 mg cm −2 . Error bars represent the standard deviations calculated from three independent measurements. Full size image After addressing the role of hydrophobicity, hydrophobic Cu-butylamine (denoted as Cu-butyl-A) without Cu 2 O was synthesized to identify the role of the Cu 2 O. Cu-butyl-A showed similar hydrophobicity (CA = 97°) with Cu/Cu 2 O-A. The XPS spectra confirmed there was no Cu 2 O in this Cu-butyl-A sample (Supplementary Figs. 20 and 21 ). At -0.7 V vs RHE, compared with that of Cu/Cu 2 O-A, Cu-butyl-A exhibited a lower FE of 84.9% for C 2 species and lower ethanol FE of 47.7% (Fig. 5 b, c and Supplementary Fig. 22 ). These results indicated the importance of Cu 2 O on promoting the C 2 products and especially on increasing the selectivity of ethanol during the CORR. This urged us to study the possible mechanism of the Cu 2 O enhancing the selectivity of ethanol by theoretic calculation. Density functional theory calculations It was reported that different facets of Cu 2 O could greatly affect the electrocatalysis performances [37] , [38] . Since the Cu 2 O (111) was clearly observed in hydrophobic Cu/Cu 2 O sample (no other facets were evidenced), we investigated the feasibility of ethanol formation on the stoichiometric oxygen-terminated (111) surface of Cu 2 O by using the density functional theory (DFT) calculations. The Gibbs free energy profile for the proposed mechanism was modeled within DFT, employing computational hydrogen electrode (CHE) approach [39] to account for the electrode potential -0.70 V vs RHE. The considered (111) surface comprises under-coordinated Cu cus atoms, which is important for the adsorption of carbon-containing intermediate species. The energy of adsorption on the (111) Cu 2 O surface is particularly favorable for the hydrogen-rich intermediates, such as *C 2 OH, *C 2 H 2 O, *C 2 H 3 O and *C 2 H 5 O. In particular, Cu cus sites are important for stabilizing these species through the interaction with non-polar carbon C, to which H atoms are progressively attached. The detailed DFT calculation information and discussion is shown in supplementary information (Supplementary Figs. 23 , 24 ). It should be noted that except the experimental observations, the DFT calculations also suggest the partial reduction of Cu 2 O surface is hindered by the presence of nBu-NH 2 , while the total reduction is completely unfavorable even at the low chemical potential of water (Supplementary Table 5 and Supplementary Figs. 25 , 26 ). In summary, hydrophobic Cu/Cu 2 O prepared through a facile one-pot synthesis method showed good selectivity for CO electroreduction into C 2 species (93.5% FE) in 2.0 M KOH electrolyte. The FE of ethanol (68.8%) ranked this material among the most efficient catalysts for electroreduction of CO 2 /CO. This hydrophobic catalyst exhibited good stability in C 2+ FE for operating over 100 hours. On the basis of the experimental results and the DFT calculation, it is concluded that suitable hydrophobicity and exposure of Cu 2 O (111) were the governing factors of CO electroreduction selectivity and stability. We anticipate that the route of this work has promising potential for converting CO into ethanol in a more selective and energy-efficient way. We also believe that the protocol to modify surface hydrophobicity can be used to prepare other efficient electrocatalysts. Synthesis of hydrophobic Cu/Cu 2 O (denoted as Cu/Cu 2 O-A) In a typical synthesis of hydrophobic Cu/Cu 2 O, 500 mg Cu(acac) 2 was added into a solution of 100 mL dimethylformamide (DMF). After vigorous stirring for 5 min, 20 mL H 2 O containing 50 mg glucose, 30 mg hexadecyl trimethyl ammonium bromide (CTAB), 110 mg polyvinyl pyrrolidone (PVP) and 5 mL n-butylamine was added by dropwise with vigorous stirring. After half an hour, the mixture was transferred into a 200 mL Teflon-lined autoclave, sealed and heated at 160 °C for 10 h. Then the system was allowed to cool down to room temperature naturally, and the mixture was collected by centrifuging, washing with ethanol and cyclohexane, and finally dried in vacuum for future characterization. Synthesis of highly hydrophobic and hydrophilic Cu/Cu 2 O (denoted as Cu/Cu 2 O-S and Cu/Cu 2 O-H, respectively) As for the synthesis of highly hydrophobic and hydrophilic Cu/Cu 2 O, the experimental process is similar to that hydrophobic Cu/Cu 2 O, except only 15 mL n-butylamine and 1 mL n-butylamine were used, respectively. Synthesis of hydrophobic Cu-butyl-A 20 mg hydrophobic Cu/Cu 2 O was placed in a quartz tube and heated to 120 °C at a flow of 5 °C min −1 under H 2 /Ar flow (V/V = 5:95) and kept at this temperature for 2 hours, then cooled down to room temperature. The powder was transferred into a solution containing 100 mL DMF, 20 mL H 2 O and 5 mL n-butylamine and stirred for half an hour. Lastly, the mixture was transferred into a 200 mL Teflon-lined autoclave, sealed and heated at 160 °C for 10 h. Then the system was allowed to cool down to room temperature naturally, and the mixture was collected by centrifuging, washing with cyclohexane, and finally dried in vacuum for future characterization. Preparation of electrode To construct the electrode, the catalyst ink was prepared by dispersing 20 mg of Cu/Cu 2 O and 80 μL of 5 wt% Nafion solution into 1 mL of water/ethanol (V/V = 4:1) solution with 3 h of sonication, and 0.1 mL of the catalyst ink was loaded on a carbon fiber paper (the gas diffusion layer, YSL-30T, 1 cm × 2 cm). Electrocatalytic analysis The CO electroreduction performances were implemented with a three-compartment electrochemical flow cell (Supplementary Fig. 7 ) connected to an electrochemical workstation (CHI760e). The as-prepared electrode, Ag/AgCl (saturated KCl) and nickel foam were used as the working electrode, reference electrode and anode, respectively. A total of 30 mL of KOH solution (0.5 M, 1.0 M, or 2.0 M) was applied as the electrolyte at both the cathode and anode sides and the cathode and anode chambers were separated by an anion exchange membrane (FFA-3, Fumatech) and the electrolytes were circulated by peristaltic pumps at the flows of 5 mL min −1 . The CO gas was introduced into the cathode with flow rate was 20 mL min −1 controlled using a mass flow controller (SevenStar D07-7). CO could diffuse into the interface between the cathode and electrolyte. All potentials were measured against the Ag/AgCl reference electrode (saturated KCl). The gas-phase products were analyzed from the outlet of the CO chamber connecting to a gas chromatography (GC) during electrolysis, and the liquid- phase products were analyzed from the electrolyte post-reaction using 1 H NMR. The Faradaic efficiency (FE) was calculated based on the Eq. ( 1 ) [4] . FE(%)=n_product×n_electron× F/ Q× 100%
 (1) where n product is the amount of the product (mol), n electron is the number of electrons transferred from CO/H 2 O into products, F is the Faradaic constant (C mol −1 ). ∆Q is the total amount of the charge that changes during the reaction. Potentials were converted to the RHE using \(E\left({{{{{\rm{RHE}}}}}}\right)=E\left({{{{{\rm{Ag}}}}}}|{{{{{\rm{AgCl}}}}}}\right)+0.197+{pH}\times 0.0591\) . The ohmic-drop correction of the potentials applied was carried out manually using the resistance measured by the electrochemical impedance spectroscopy under open circuit potentials once the electrolysis was completed. All of the electrocatalytic reactions were implemented at ambient pressure and temperature and 85% ohmic resistance correction was applied in all the measurements. The gas products were collected and analysed every 10 or 30 min during the reaction. DFT calculation All calculations have been performed within the Density Functional theory (DFT) applying PBE functional [40] . The absorption studies on the Cu 2 O surface were carried out using Quantum Espresso ab initio simulation package [41] . The non-polar oxygen-terminated stoichiometric (111) surface of Cu 2 O was cut out from a cubic bulk Cu 2 O structure with 4.301 Å lattice parameter obtained by full geometry relaxation with PBE functional. The constructed 3-layer 1×1 surface, comprising 18 atoms, with a = b = 6.082 Å lattice parameters and more than 20 Å of vacuum in z-direction was relaxed at DFT-PBE level. The structures of all surfaces with intermediate adsorbates were also fully relaxed. All adsorbates are assumed to be neutral species. All these calculations employed a plane wave basis set with 80 Ry and 640 Ry kinetic energy and charge density cutoffs, respectively. Core electrons were described with Vanderbuilt ultrasoft pseudopotentials [42] . A 2×2×1 Γ-centered k-point mesh was employed. The temperature contribution into ΔG was accounted by calculating vibrational contributions (ZPE, H, S) for adsorbates and vibrational, translational and rotational contributions for desorbed species within the ideal gas model, using CP2K code [43] . The consecutive electro-reduction of CO was modelled using Computational Hydrogen Electrode (CHE) approach [39] , employing reversible hydrogen electrode (RHE) as a reference. Materials characterization Fourier transform infrared (FT-IR) spectra were recorded on an Advatar 380 Thermo Nicolet (America) in transmission mode at a resolution of 4 cm −1 . Elemental analysis was carried out with a CE instruments EA 1110 elemental analyzer (PerkinElmer, America). Thermogravimetric analysis (TGA) was operated on a TA Q500 instrument (America) under nitrogen atmosphere. Powder X-ray diffraction (XRD) patterns were recorded on a Rigaku Ultima IV powder X-ray diffractometer (Japan) (Cu Kα, λ = 1.54184 Å) at room temperature. X-ray photoelectron spectroscopy (XPS) spectra were recorded on a Thermo Escalab 250Xi spectrometer (America) using a photon energy of 461 eV with an energy resolution of 0.1 eV. Transmission electron microscopy (TEM) was carried out on a JEM 1400 under 200 KV. The X-ray absorption spectroscopy (XAS) measurements were performed using the QEXAFS configuration on the SuperXAS beamline (at the SLS, Villigen) [44] . The storage ring operated at 2.4 GeV in top-up mode with a ring current of 400 mA, and a focal spot size on the sample position was of 500 × 200 μm( H × V ). The measurements were performed in the traditional transmission geometry using ion-chambers; the data extraction and processing were performed by using ProQEXAFS and the beamline dedicated XAS analysis software [45] . For increased S/N, the data was subsequently averaged over a 600 s total acquisition per sample. Finally, Demeter package (Athena/Artemis) was used for further post-processing and fitting [46] . GC analysis GC was carried out on a FuLi instruments GC9790II with the Ar carrier gas. The thermal conductivity detector (TCD) was used to quantify H 2 concentration and all the carbon-based products were detected using the flame ionization detector (FID) with a methanizer. The detectors are calibrated by two independent standard gases. 1 H-NMR spectroscopy 1 H-nuclear magnetic resonance spectroscopy ( 1 H-NMR) was performed on a Bruker AC-600 MHz instrument (Switzerland). Typically, 0.5 mL of electrolyte after electrolysis was mixed with 0.1 mL of D 2 O (Sigma-Aldrich, purity: 99.9%) containing 100 ppm dimethyl sulfoxide (DMSO, Sigma-Aldrich, 99.9%) as the internal standard. To ensure the accuracy, both the standard method and external method were employed to calculate the liquid products and the results were exhibited in Supplementary Figs. 27 , 28 and Supplementary Table 6 . Carbon balance To elucidate the carbon balance path, flow meters were used to monitor the inlet and outlet flow out of the reactor and the results were showed in Supplementary Fig. 29 and Supplementary Table 7 . In-situ Raman studies In-situ Raman spectra acquisition was performed using a Renishaw confocal Raman system with the laser excitation at 532 nm. The laser power is kept at 1.5 mW to protect the sample from laser damage. Cu/Cu 2 O-A catalyst was spread on the glassy carbon connecting an external metal bar, which is used as the working electrode that contacts only CO-saturated electrolyte. The other metal bar connecting with a platinum wire extending in the cell was used as the counter electrode. An Ag/AgCl electrode was used as the reference electrode. 2.0 M KOH electrolyte was poured into the cell to immerse these electrodes. The collection time was 10 s and repeated for 3 times for the Cu/Cu 2 O-A sample. The CORR test was performed at the potential of -1.77 V vs Ag/AgCl and a computer synchronously collected the Raman signals. 13 CO electrolysis The experiment was performed with labeled 13 CO gas (99.0%, Sigma Aldrich) for electrolysis. The 13 CO gas flow rate was controlled using a mass flow controller (SevenStar D07-7) at a rate of 20 mL min −1 . 13 CO electroreduction was conducted at a constant current of 160 mA cm −2 for 10 min and the gas products and the catholyte were collected for analysis by gas chromatography-mass spectrometry (GC-MS).